Biocatalytic trifluoromethylation of unprotected phenols Organofluorine compounds have become important building blocks for a broad range of advanced materials, polymers, agrochemicals, and increasingly for pharmaceuticals. Despite tremendous progress within the area of fluorination chemistry, methods for the direct introduction of fluoroalkyl-groups into organic molecules without prefunctionalization are still highly desired. Here we present a concept for the introduction of the trifluoromethyl group into unprotected phenols by employing a biocatalyst (laccase), t BuOOH, and either the Langlois’ reagent or Baran’s zinc sulfinate. The method relies on the recombination of two radical species, namely, the phenol radical cation generated directly by the laccase and the CF 3 -radical. Various functional groups such as ketone, ester, aldehyde, ether and nitrile are tolerated. This laccase-catalysed trifluoromethylation proceeds under mild conditions and allows accessing trifluoromethyl-substituted phenols that were not available by classical methods. The introduction of fluoroalkyl-groups (for example, CF 3 , CHF 2 , CH 2 F, etc.) into organic compounds has become a major subject in various fields of chemical research, in particular medicinal chemistry and drug discovery [1] , [2] . This is due to the metabolic stability, increased permeability or enhanced binding properties of the organo-fluorine compounds in comparison to their non-fluorinated counterparts [3] . Among all fluorine-containing moieties, the trifluoromethyl group is privileged [4] , and trifluoromethylated arenes are of interest for agrochemicals, pharmaceuticals and advanced materials [5] . Several excellent methods to provide structurally diverse CF 3 -building blocks have been elaborated [6] , [7] , [8] : common strategies to introduce the CF 3 -group into aromatic compounds involve metal-mediated/catalysed functional group interconversions [9] , [10] where halogens [11] , [12] , [13] , boronic acids [14] , [15] , [16] , boronates [17] , [18] and even amines [19] , [20] are replaced by nucleophilic, electrophilic or radical CF 3 -sources ( Fig. 1a ). Other methods rely on directing groups [21] , [22] , [23] , as well as on visible light and photo-catalysis ( Fig. 1b,c ) [24] , [25] , [26] . 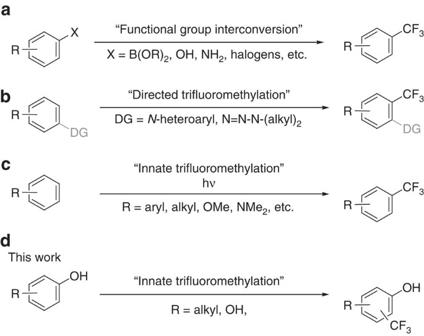Figure 1: Methods to attach the CF3-group to arenes. (a) Functional group interconversion; (b) Trifluoromethylation controlled by a directing group (DG); (c) Innate trifluoromethylation of substituted arenes, accept phenols; (d) Innate trifluoromethylation of phenols. Figure 1: Methods to attach the CF 3 -group to arenes. ( a ) Functional group interconversion; ( b ) Trifluoromethylation controlled by a directing group (DG); ( c ) Innate trifluoromethylation of substituted arenes, accept phenols; ( d ) Innate trifluoromethylation of phenols. Full size image While trifluoromethylation of (substituted) mono- and biaryl-systems has been broadly investigated [27] , [28] , [29] , [30] , only few reports deal with the transformation of unprotected phenols ( Fig. 1d ) [31] , [32] , [33] , and these give non-regioselective transformations and/or unsatisfying conversions. Hence, a general method for attaching the CF 3 -moiety to phenols in a practical manner remains elusive. We report an efficient and selective method for trifluoromethylation of unprotected phenols by biocatalytic introduction of a trifluoromethyl group derived from common precursors. Reaction concept The approach for the trifluoromethylation of phenols via C–C bond formation presented in this paper is based on the recombination of two radicals, namely a CF 3 -radical and a phenol-derived radical, wherein the two radicals are formed via two different pathways ( Fig. 2 ). The phenol-derived radical is formed by a laccase (E.C. 1.10.3.2), which catalyses in general the one-electron oxidation of phenols and anilines using molecular oxygen as the oxidant [34] , [35] , [36] , [37] , [38] . Simultaneously, the electrophilic CF 3 -radical is generated in situ from either Langlois’ reagent (NaSO 2 CF 3 ) [31] , [39] , [40] or Baran’s zinc sulfinate (Zn(SO 2 CF 3 ) 2 =TFMS) [41] . The CF 3 -radical may also be formed under electrochemical conditions from TFMS [42] . 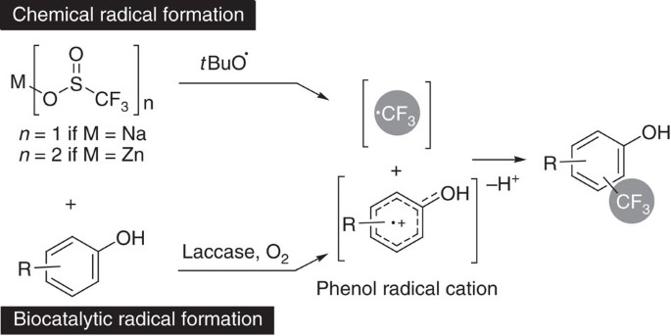Figure 2: Biocatalytic trifluoromethylation of unprotected phenols. Radical trifluoromethylation of unprotected phenols by recombination of radicals generated via two different pathways. Figure 2: Biocatalytic trifluoromethylation of unprotected phenols. Radical trifluoromethylation of unprotected phenols by recombination of radicals generated via two different pathways. Full size image The concept was initially tested by employing the laccase from Agaricus bisporus and using the electron-rich phenol 1a as substrate and TFMS as trifluoromethylation agent with tert- butyl hydroperoxide ( t BuOOH) as the oxidant. This ortho- and para-substituted substrate was chosen to minimize literature-known fast di- or oligomerization in ortho and para positions initiated by laccases [34] , [35] , [36] , [37] , [43] . The chemical-enzymatic system led to successful product formation, whereby O-alkylation was not detected, but C–C bond formation at the free C–H of the arene was observed, leading to product 2a with 58% of the transformed substrate ( Table 1 , entry 1). Table 1 Laccase-mediated trifluoromethylation of unprotected phenols in combination with TFMS. Full size table The phenol did not react in the absence of laccase and in the presence of TFMS and t BuOOH (Entry 2). In the presence of the laccase but in the absence of TFMS/ t BuOOH, substrate 1a was just di-/polymerized (Entry 3). Also, performing the reaction with laccase and TFMS in the absence of t BuOOH did not lead to the desired product formation of 2a , indicating that t BuOOH is required to form the CF 3 -radical (Entry 4). Thus, product 2a was only formed in the presence of laccase and TFMS/ t BuOOH. t BuOOH cannot be substituted by hydrogen peroxide, since in this case neither the formation of trifluoromethylated 2a nor any other transformation of 1a was observed (entry 5). Encouraged by this initial result, the radical trifluoromethylation of 1a was optimized, testing varied concentrations of TFMS, t BuOOH, co-solvents as well as temperature (see Supplementary Information ). The best conditions for the formation of 2a were found at 50 mM phenol 1a with 2.0 eq. TFMS and 8.0 eq. t BuOOH at 30 °C in the presence of 25 vol% dimethylsulfoxide (DMSO). Functional group tolerance To tap the scope and functional group tolerance of this method, various substituted phenols 1a-h were transformed under optimized conditions, whereby the ortho- and para-position with respect to the phenolic hydroxyl moiety were blocked for substrate 1a - c ( Table 2 ). In these cases, products 2a - c with the CF 3 -moiety meta to the OH were isolated with exquisite regio-control (entry 1–3), and for 2b and 2c also verified by X-ray crystallography ( Fig. 3 ). Comparable results were obtained independent of the trifluoromethylation agent employed: thus, the Langlois’ reagent as well as the Baran’s zinc sulfinate led to comparable isolated yields up to 62%. Moreover, the reaction system tolerated ketone-, ester-aldehyde, as well as nitrile-functionalities, emphasizing the mildness of the reaction. Interestingly, nitrogen-containing substrates like indol or 4-aminoacetophenone were not converted at all under the reaction conditions investigated, while other substrates like sesamol, 5,6,7,8-tetrahydro-2-naphthol, 2-naphthol or meta-dimethylamino acetophenone resulted in complex product mixtures. Table 2 Scope and functional group tolerance of the biocatalytic trifluoromethylation of unprotected phenols employing Baran’s zinc sulfinate or Langlois’ reagent in combination with a laccase. 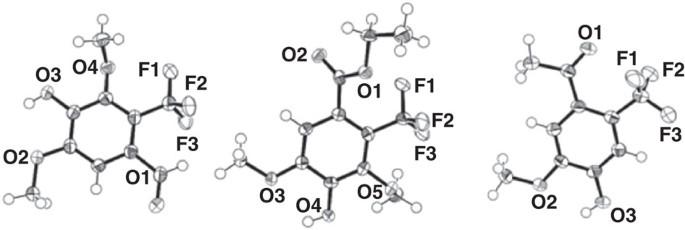Figure 3: Crystal structures of 2b, 2c and 2d-meta. Stereoscopic ORTEP plot of crystals2b,2cand2d-meta. The probability ellipsoids were drawn on 50% probability. Radii of hydrogen atoms are drawn arbitrarily. Full size table Figure 3: Crystal structures of 2b, 2c and 2d- meta . Stereoscopic ORTEP plot of crystals 2b , 2c and 2d - meta . The probability ellipsoids were drawn on 50% probability. Radii of hydrogen atoms are drawn arbitrarily. Full size image Regioselectivity The transformation of phenols 1d and 1e , bearing only a single substituent ortho to the phenolic hydroxy group, led to a mixture of regio-isomers, albeit with significant preference for the meta-isomers (C2:C3=4:1 up to 10:1, entry 4 and 5). The preferred meta-substitution for 2d was confirmed via a crystal structure ( Fig. 3 ). It is worth noting that substrate 1f , being devoid of ortho-methoxy substituents, afforded only the isomer bearing the CF 3 moiety ortho to the alcohol group with 31% isolated yield (entry 6). In a similar fashion, substrate 1g possessing in para position a nitrile group instead of the acetyl moiety resulted in the mono-substituted ortho-product 2g with 57% isolated yield (entry 7). Taking a substrate devoid of a para-substituent but having methoxy substituents in both ortho positions ( 1h ), the trifluoromethylation protocol led to a di-trifluoromethylated product, 2h , having a CF 3 -group in ortho as well as meta position with respect to the phenolic OH (entry 8). The observed regioselectivity for 2d - f can be explained by the transition state energies of the addition of the CF 3 -radical to the phenol radical cations. For instance, the corresponding transition state leading to 2d with substitution at C2 is energetically preferred over substitution at C3 (2.1 kcal mol −1 , M06-2X/6-311+G(d,p)) ( Fig. 4 , Supplementary Fig. 5 ). The same is true for the analogous transition state leading to 2e ( Supplementary Fig. 6 ). The energies of the substituted intermediate cations after addition of the CF 3 -radical to the phenol radical cation also reflect the observed regioselectivity. In the case of substrate 1f , the energies of the transition states support the expected and observed substitution in ortho-position to the phenolic OH leading to product 2f ( Supplementary Fig. 6 ). Since the energies of the transition states reflect the observed regioselectivity, the bio-trifluoromethylation is mainly not active site-directed. 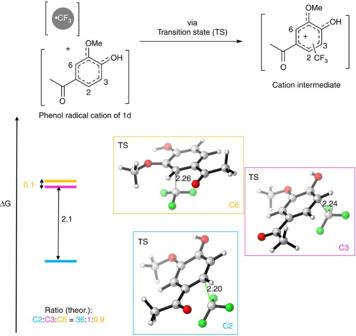Figure 4: Energy differences of transition states. Energy differences and structures of transition states leading preferentially to substitution at C2 giving2d. Figure 4: Energy differences of transition states. Energy differences and structures of transition states leading preferentially to substitution at C2 giving 2d . Full size image Mechanism The computational calculations also showed that the CF 3 -radical has to react preferentially with the phenol radical cation and not with the corresponding already deprotonated phenoxy radical, since the latter would lead, for example, for 1d , to substitution in ortho-position to the hydroxy group and not at the mainly observed meta-position. Substitution in ortho-position would be favoured over meta-position by 3 kcal mol −1 upon combination with the neutral phenoxy radical. Therefore, in the proposed mechanism the laccase oxidizes the phenol 1d via a single electron transfer to the phenol radical cation ( Fig. 5 ). The latter reacts with the CF 3 -radical to give the cationic intermediate, which rearomatizes to the final product. As shown in the initial experiments, trifluoromethylation only occurred in the presence of laccase and TFMS/ t BuOOH ( Table 1 , entry 1); the phenol starting material did not react with TFMS/ t BuOOH (entry 2), nor did the phenol radical cation (formed by laccase and O 2 present) react with TFMS (entry 4). 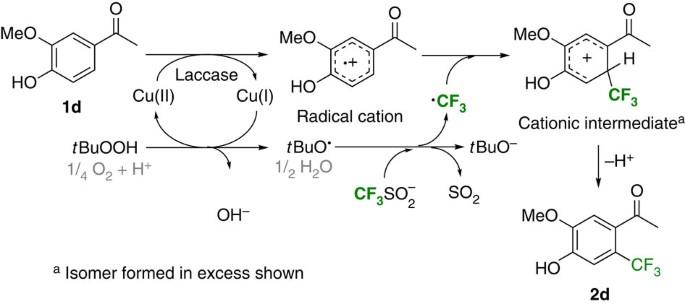Figure 5: Proposed mechanism for laccase-catalysed trifluoromethylation of phenols. Proposed mechanism for the laccase-mediated trifluoromethylation of unprotected phenols exemplified for substrate1d. For reasons of clarity the scheme displays only the productive pathway relevant for the formation of2b; other reactions, for example, like HCF3formation, dimerization of the CF3-radical or the radical cation, the decay oftBuOOH and the oxidation of SO2are omitted, as well as the formation of minor regio-isomers. Figure 5: Proposed mechanism for laccase-catalysed trifluoromethylation of phenols. Proposed mechanism for the laccase-mediated trifluoromethylation of unprotected phenols exemplified for substrate 1d . For reasons of clarity the scheme displays only the productive pathway relevant for the formation of 2b ; other reactions, for example, like HCF 3 formation, dimerization of the CF 3 -radical or the radical cation, the decay of t BuOOH and the oxidation of SO 2 are omitted, as well as the formation of minor regio-isomers. Full size image In the recently proposed mechanism [39] , traces of redox metals are proposed to initiate the reaction for the first transformation of t BuOOH to t BuO· and OH − . t BuO· enables the formation of the CF 3 · species. In the reported catalytic cycle the activation of t BuOOH was triggered by the heteroaromatic radical intermediates. Since in the laccase-catalysed trifluoromethylation of phenol, the laccase provides already one reactive radical species for the C–C bond forming reaction, namely the phenol radical cation, stoichiometric amounts of redox metal (for example, Fe, Co, Cu mentioned in previous work) would be required to obtain the amount of t BuO· needed. Since the trifluoromethylation went to high conversion without addition of any metals or other redox reagents, it was deduced that the copper Cu(I) present in the laccase also reacts with t BuOOH to give t BuO· and Cu(II) as already proposed in previous papers using only Cu (ref. 31 ). This was also supported by photometric assays in laccase-catalysed oxidative dimerization of 2,6-dimethoxy phenol showing that the presence of t BuOOH led to a faster reaction ( Supplementary Methods , Photometric Enzymatic Activity Assay). Thus, the Cu(I) of the laccase can be oxidized by t BuOOH, which leads to t BuO· as previously reported [31] ; the latter reacts with the CF 3 SO 2 − to set free the CF 3 -radical, as proven elsewhere [39] . Comparison to literature methods To compare the here-presented laccase/ t BuOOH protocol with published methods for the chemical trifluoromethylation of (electron-rich) arenes and hetero-arenes [29] , [30] , phenols 1a (R=Me) and 1b (R=H) were treated with Ruppert-Prakash reagent [44] TMSCF 3 in the presence of catalytic silver (AgF) and PhI(OAc) 2 as oxidant ( Fig. 6a ). 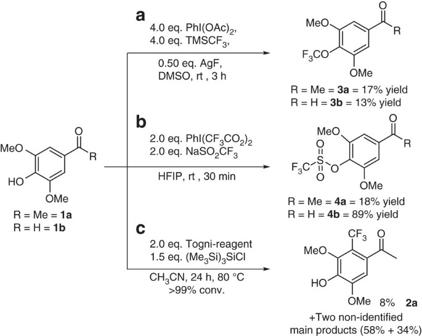Figure 6: Methods from literature tested for comparison. Trifluoromethylation methods for electron-rich arenes for comparison with the here-presented laccase/tBuOOH concept. (a) Method involving silver as metal; metal-free trifluoromethylations using phenyl-iodine bis(trifluoroacetate) (b) or Togni-reagent (c). Figure 6: Methods from literature tested for comparison. Trifluoromethylation methods for electron-rich arenes for comparison with the here-presented laccase/ t BuOOH concept. ( a ) Method involving silver as metal; metal-free trifluoromethylations using phenyl-iodine bis(trifluoroacetate) ( b ) or Togni-reagent ( c ). Full size image For both substrates 1a and 1b only minor amounts of 2a and 2b were found in a complex product mixture; the major product components were the trifluoromethyl-aryl-ethers 3a and 3b (13–17% isolated yield). A related CF 3 -ether formation was reported recently [45] . As a second literature method a metal-free alternative for the trifluoromethylation of arenes and biaryls was investigated [30] , whereby the CF 3 -radical is generated by the oxidation of the Langlois’ reagent NaSO 2 CF 3 with phenyl-iodine bis(trifluoroacetate) ( Fig. 6b ). In this case the transformation of 1a and 1b led to the corresponding trifluoromethanesulfonates 4a and 4b as the main products (18–89% isolated yield), while 2a and 2b (R=H) were found only in negligible quantities. As a third method the Togni reagent [32] , [46] was employed for substrate 1a ( Fig. 6c ); although the substrate was completely converted, product 2a was only a minor product (8%), while two non-identified main products were detected, which did not contain any CF 3 -group. Thus, the laccase trifluoromethylation reported here is clearly complementary to literature methods tested. With this study, we have achieved radical C–CF 3 bond formation by the recombination of two radical species—one generated biocatalytically and the other in a chemical reaction. This method represents the first biocatalyst-dependent trifluoromethylation of organic compounds, especially unprotected phenols, giving access to building blocks that were not accessible as major products by any other method described before. Moreover, the methods display a high functional group tolerance, allowing the conversion of aldehydes, esters and ketones without decomposition, which makes this method suitable for late-stage trifluoro-methylations. The method proceeds under mild reaction conditions with high regioselectivity. Representative trifluoromethylation procedure (1 ml) The laccase from A. bisporus (7.5 U, 5.0 mg ml −1 final conc.) was dissolved in a sodium acetate buffer (695 μl, 250 mM, pH 5.5) prior to addition of Zn(SO 2 CF 3 ) 2 (2 eq., 33.2 mg dissolved in DMSO). Afterwards ketone 1 (50 mM final concentration, dissolved in DMSO) was added followed by aqueous t BuOOH solution (8.0 eq., 55 μl, 70 wt% aqueous solution) to reach a total volume of 1.0 ml (25 vol% DMSO). The reactions were shaken in an orbital shaker at 30 °C (Zn(SO 2 CF 3 ) 2 ) or 40 °C in case of NaSO 2 CF 3 for 24 h at 900 r.p.m. (horizontal position). Then, each 1 ml reaction was extracted four times with EtOAc (500 μl) and combined organic fractions were dried over Na 2 SO 4 . The solutions were filtered, concentrated under reduced pressure and the residue was purified by various solvent mixtures to afford the trifluoromethylated phenol derivative 2. QM calculations Full geometry optimizations, transition structure searches and single-point computations were carried out with the Gaussian 09 package [47] . All geometry optimizations were carried out with the unrestricted version of the hybrid B3LYP functional [48] . For C, O, N and H, the double-zeta basis set 6–31G(d) was employed to obtain the geometries, and the larger 6–311+G(d,p) basis set was used to calculate single-point energies. Additional single-point energy calculations using functionals able to account for dispersion forces such as M06-2X (ref. 49 ) in conjunction with the 6–311+G(d,p) basis set were performed ( Supplementary Table 5 ). Thermal and entropic corrections to energy were calculated from vibrational frequencies. The nature of the stationary points was determined in each case according to the appropriate number of negative eigenvalues of the Hessian matrix from the frequency calculations. Frequencies were not scaled. Data availability Crystal structures that support the findings of this study have been deposited at the Cambridge Crystallographic Data Centre and allocated the deposition numbers CCDC 1480621 ( 2b ), 1480623 ( 2c ) and CCDC 1480622 ( 2d ). All other data supporting the findings of this study are available within the article and its Supplementary Information file or from the author upon reasonable request. How to cite this article: Simon, R. C. et al . Biocatalytic trifluoromethylation of unprotected phenols. Nat. Commun. 7 , 13323 doi: 10.1038/ncomms13323 (2016). Publisher's note: Springer Nature remains neutral with regard to jurisdictional claims in published maps and institutional affiliations.